Extracellular Ca2+is a danger signal activating the NLRP3 inflammasome through G protein-coupled calcium sensing receptors Activation of the NLRP3 inflammasome enables monocytes and macrophages to release high levels of interleukin-1β during inflammatory responses. Concentrations of extracellular calcium can increase at sites of infection, inflammation or cell activation. Here we show that increased extracellular calcium activates the NLRP3 inflammasome via stimulation of G protein-coupled calcium sensing receptors. Activation is mediated by signalling through the calcium-sensing receptor and GPRC6A via the phosphatidyl inositol/Ca 2+ pathway. The resulting increase in the intracellular calcium concentration triggers inflammasome assembly and Caspase-1 activation. We identified necrotic cells as one source for excess extracellular calcium triggering this activation. In vivo , increased calcium concentrations can amplify the inflammatory response in the mouse model of carrageenan-induced footpad swelling, and this effect was inhibited in GPRC6A −/− mice. Our results demonstrate that G-protein-coupled receptors can activate the inflammasome, and indicate that increased extracellular calcium has a role as a danger signal and amplifier of inflammation. The multi-protein complex of the NLRP3 inflammasome is assembled in response to danger-associated stimuli during infectious [1] or sterile [2] inflammatory events, but the involved proximal signalling pathways are only partially characterized. Extracellular calcium concentrations (ex[Ca 2+ ]) are tightly regulated in the extracellular interstitial fluid and presumed to range from 0.9 to 1.2 mM [3] , [4] . The ex[Ca 2+ ] concentrations are known to be increased at sites of infections [5] , [6] and in the interstitial fluid around activated cells [7] , but the resulting cellular consequences are not known. The presence of calcifications at sites of chronic inflammation or ischaemic necrosis [8] , [9] suggests, however, that ex[Ca 2+ ] can increase not only in infectious but also in sterile inflammation. We hypothesized, therefore, that increased ex[Ca 2+ ] conveys a danger signal to surrounding cells and triggers inflammasome activation. Here we show that increased extracellular calcium concentrations result in an amplification of inflammatory responses, which can be inhibited by antagonists of calcium-sensing receptor (CaSR), and which is significantly reduced in monocytes from GPRC6A −/− mice. ex[Ca 2+ ] induces IL-1β through the NLRP3 inflammasome To test the hypothesis that extracellular calcium triggers inflammasome activation, monocytes were stimulated in vitro with increasing ex[Ca 2+ ]. 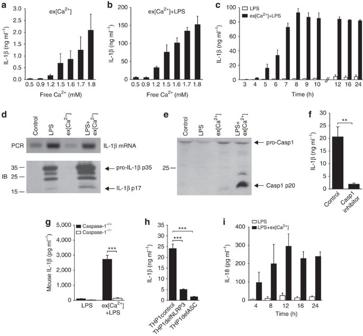Figure 1: Extracellular calcium induces monocyte IL-1β release by activating the inflammasome. (a,b) IL-1β release of CD14+ monocytes in response to increasing ex[Ca2+] alone (a) or to increasing ex[Ca2+] plus LPS (b) after 16 h of stimulation (n=3). (c) time course of IL-1β release of CD14+ monocytes after stimulation with LPS alone or with increased ex[Ca2+] (1.7 mM) plus LPS (n=3). (d) PCR (upper panel) and immunoblot (IB, lower panel) for IL-1β in unstimulated monocytes (control) and in monocytes stimulated with LPS, with increased ex[Ca2+] concentration (1.7 mM), or both, after 16 h of culture. Specific bands for IL-1β mRNA, pro-IL-1β p35 and IL-1β p17 as indicated. One representative experiment out of three is shown. (e) IB analysis of Caspase-1, which shows the activation of Caspase-1 in supernatants harvested from unstimulated monocytes (control) and in monocytes stimulated with LPS, with increased ex[Ca2+] concentration (1.7 mM), or with both, after 16 h of culture. Specific bands for pro-Caspase-1 (pro-Casp1) and Caspase-1 (Casp1 p20) are indicated, shown is one representative blot out of three experiments performed. (f) IL-1β secretion of monocytes stimulated with ex[Ca2+] plus LPS in the absence and presence of the caspase-1 inhibitor Z-WEHD-FMK (5 μM,n=3). (g) mIL-1β secretion of monocytes from Caspase-1+/+and Caspase-1−/−NOD mice stimulated with LPS or with ex[Ca2+] plus LPS (n=3). (h) IL-1β secretion of THP-1 cells (control), NLRP3-deficient THP-1 cells (THP1defNLRP3) and ASC-deficient THP-1 cells (THP1defASC) stimulated with increased ex[Ca2+] concentration (1.7 mM) and LPS, after 16 h of culture (n=3). (i) Time course of IL-18 release of CD14+ monocytes after stimulation with LPS alone or with increased ex[Ca2+] (1.7 mM) plus LPS (n=3). In all experiments, cytokine concentrations were determined in the supernatant by enzyme-linked immunosorbent assay. All bars show mean±s.e.m. Statistical analysis was performed using the two-tailed Student’st-test; **P<0.01 and ***P<0.001. To raise the concentration of free calcium ions in serum-supplemented tissue culture media, CaCl 2 had to be added in excess (for titration, see Supplementary Table 1 ). After 16 h, a concentration-dependent increase in ex[Ca 2+ ]-induced IL-1β secretion was detected ( Fig. 1a ). Figure 1: Extracellular calcium induces monocyte IL-1β release by activating the inflammasome. ( a , b ) IL-1β release of CD14+ monocytes in response to increasing ex[Ca 2+ ] alone ( a ) or to increasing ex[Ca 2+ ] plus LPS ( b ) after 16 h of stimulation ( n =3). ( c ) time course of IL-1β release of CD14+ monocytes after stimulation with LPS alone or with increased ex[Ca 2+ ] (1.7 mM) plus LPS ( n =3). ( d ) PCR (upper panel) and immunoblot (IB, lower panel) for IL-1β in unstimulated monocytes (control) and in monocytes stimulated with LPS, with increased ex[Ca 2+ ] concentration (1.7 mM), or both, after 16 h of culture. Specific bands for IL-1β mRNA, pro-IL-1β p35 and IL-1β p17 as indicated. One representative experiment out of three is shown. ( e ) IB analysis of Caspase-1, which shows the activation of Caspase-1 in supernatants harvested from unstimulated monocytes (control) and in monocytes stimulated with LPS, with increased ex[Ca 2+ ] concentration (1.7 mM), or with both, after 16 h of culture. Specific bands for pro-Caspase-1 (pro-Casp1) and Caspase-1 (Casp1 p20) are indicated, shown is one representative blot out of three experiments performed. ( f ) IL-1β secretion of monocytes stimulated with ex[Ca 2+ ] plus LPS in the absence and presence of the caspase-1 inhibitor Z-WEHD-FMK (5 μM, n =3). ( g ) mIL-1β secretion of monocytes from Caspase-1 +/+ and Caspase-1 −/− NOD mice stimulated with LPS or with ex[Ca 2+ ] plus LPS ( n =3). ( h ) IL-1β secretion of THP-1 cells (control), NLRP3-deficient THP-1 cells (THP1defNLRP3) and ASC-deficient THP-1 cells (THP1defASC) stimulated with increased ex[Ca 2+ ] concentration (1.7 mM) and LPS, after 16 h of culture ( n =3). ( i ) Time course of IL-18 release of CD14+ monocytes after stimulation with LPS alone or with increased ex[Ca 2+ ] (1.7 mM) plus LPS ( n =3). In all experiments, cytokine concentrations were determined in the supernatant by enzyme-linked immunosorbent assay. All bars show mean±s.e.m. Statistical analysis was performed using the two-tailed Student’s t -test; ** P <0.01 and *** P <0.001. Full size image For inflammasome-dependent IL-1β release, an initial signal via toll-like receptor (TLR) stimulation is required to increase pro-IL-1β synthesis [2] . Accordingly, lipopolysaccharide (LPS) priming of monocytes prior to stimulation with ex[Ca 2+ ] lead to a striking increase in IL-1β production ( Fig. 1b ; for other TLR ligands, see Supplementary Fig. S1 ). IL-1β secretion started 4 h after stimulation with ex[Ca 2+ ], peaked after 8 h and remained stable thereafter ( Fig. 1c ), with no discernible influence of the duration of LPS priming or the ex[Ca 2+ ] concentration during pre-incubation ( Supplementary Fig. S2a,b ). Increased ex[Ca 2+ ] had no influence on IL-1β mRNA expression, but was found to trigger proteolytic cleavage of pro-IL-1β protein into IL-1β p17 ( Fig. 1d ). Accordingly, activated Caspase-1 was detectable by western blot following stimulation with ex[Ca 2+ ] ( Fig. 1e ), whereas the Caspase-1 inhibitor Z-WEHD-FMK abrogated ex[Ca 2+ ]-induced release of IL-1β ( Fig. 1f ). Most importantly, monocytic cells from Caspase-1 −/− mice did not produce IL-1β in response to increased ex[Ca 2+ ], whereas wild-type (wt) Caspase-1 +/+ mice ( Fig. 1g ) and IL-1R −/− mice ( Supplementary Fig. S3 ) did. Evidence for inhibition of ex[Ca 2+ ]-induced IL-1β secretion by geldanamycin and high extracellular K + concentration ( Supplementary Fig. S4 ) suggested involvement of the inflammasome. This was confirmed in experiments with THP-1 cells deficient for the adaptor protein apoptosis-associated speck-like protein containing a CARD (ASC), which were found not to respond to increased ex[Ca 2+ ] ( Fig. 1h ). Similarly, NLRP3-deficient THP-1 cells also showed a greatly reduced response ( Fig. 1h ), indicating that this inflammasome is required for the monocytic response to increased ex[Ca 2+ ]. The expression of NLRP3 mRNA in human monocytes was not influenced by stimulation with LPS+ex[Ca 2+ ] ( Supplementary Fig. S5 ). The inflammasome-dependent cytokine IL-18 [10] was found to be secreted with similar kinetics as IL-1β ( Fig. 1i ). ex[Ca 2+ ] activates the inflammasome via CaSR and GPRC6A Cells sense ex[Ca 2+ ] through two G-protein-coupled receptors (GPCRs), CaSR [11] and GPRC6A [12] , [13] . Both receptors are expressed in human monocytes as confirmed by western blot ( Fig. 2a ) and quantitative reverse transcriptase PCR (qRT–PCR) (data not shown). Two selective inhibitors of CaSR and GPRC6A, Calhex231 and NPS2143 (ref. 14 ) were found to significantly decrease ex[Ca 2+ ]-induced IL-1β production ( Fig. 2b ), but had no influence on adenosine triphosphate (ATP)-induced inflammasome activation ( Supplementary Fig. S6 ). In addition, Calhex231 inhibited the ex[Ca 2+ ]+LPS-induced processing of active Caspase-1 ( Fig. 2c ). 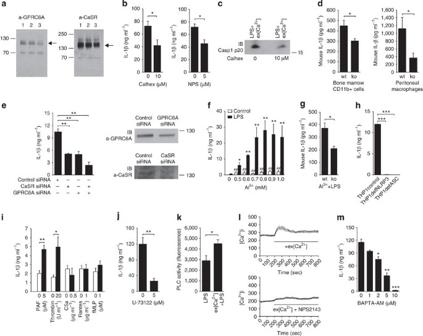Figure 2: Extracellular calcium activates the inflammasome via CaSR and GPRC6A. (a) Immunoblot (IB) analysis demonstrating the expression of GPRC6A (left panel) and CaSR (right) in human monocytes. In both blots, lanes 1, 2 and 3 represent three different healthy donors. (b) Influence of Calhex231 and NPS2143 on the IL-1β secretion of monocytes stimulated with increased ex[Ca2+]+LPS (n=3). (c) IB analysis showing the active form of caspase-1 (p20) in supernatants collected from monocytes stimulated with increased ex[Ca2+]+LPS in the absence or presence of Calhex231 after 16 h of culture. One representative blot out of three experiments performed is shown. (d) Ex[Ca2+]-induced IL-1β secretion of CD11b+ mononuclear cells isolated from bone marrow and of peritoneal macrophages from GPRC6A+/+(wt) and GPRC6A−/−(ko) mice (n=5). (e) Influence of CaSR and GPRC6A inactivation by transfection with siRNA on IL-1β secretion of THP-1 cells in response to ex[Ca2+]+LPS (n=3). IBs show inhibition of protein expression of GPRC6A and CaSR in cells transfected with the respective siRNA compared with control siRNA. (f) IL-1β secretion of monocytes in response to increasing concentration of Al3+with or without LPS (n=3). (g) IL-1β secretion of peritoneal macrophages from GPRC6A+/+(wt) and GPRC6A−/−(ko) mice in response to 0.9mM Al3+plus LPS (n=3). (h) IL-1β secretion of THP-1 cells (control), NLRP3-deficient THP-1 cells (THP1defNLRP3) and ASC-deficient THP-1 cells (THP1defASC) stimulated with 0.9 mM Al3+plus LPS, for 16 h (n=3). (i) IL-1β release of monocytes stimulated with different GPCR ligands at the indicated concentration alone (white bars) or with GPCR ligands +LPS (black bars) for 16 h. (j) IL-1β release from monocytes stimulated with ex[Ca2+]+LPS in the presence of dimethyl sulfoxide (control) or with the phosphoinositide-specific PLC inhibitor U-73122 (5 μM) in dimethyl sulfoxide (n=3). (k) PLC activity in monocytes stimulated for 16 h with LPS alone or with ex[Ca2+]+LPS (n=5). (l) For [Ca2+]iimaging, monocytes were loaded with the Ca2+-sensitive indicator dye Fura-2-AM and subsequently stimulated with ex[Ca2+] (1.7 mM). The increase in [Ca2+]iwas inhibited by NPS2143. One representative experiment out of three is shown. (m) IL-1β release from monocytes stimulated with ex[Ca2+]+LPS in the presence of increasing concentrations of BAPTA-AM (n=3). *P<0.05, **P<0.01 and ***P<0.001, always in comparison with the negative control. Statistical analysis was performed using the two-tailed Student'st-test. All error bars show mean±s.e.m. Figure 2: Extracellular calcium activates the inflammasome via CaSR and GPRC6A. ( a ) Immunoblot (IB) analysis demonstrating the expression of GPRC6A (left panel) and CaSR (right) in human monocytes. In both blots, lanes 1, 2 and 3 represent three different healthy donors. ( b ) Influence of Calhex231 and NPS2143 on the IL-1β secretion of monocytes stimulated with increased ex[Ca 2+ ]+LPS ( n =3). ( c ) IB analysis showing the active form of caspase-1 (p20) in supernatants collected from monocytes stimulated with increased ex[Ca 2+ ]+LPS in the absence or presence of Calhex231 after 16 h of culture. One representative blot out of three experiments performed is shown. ( d ) Ex[Ca 2+ ]-induced IL-1β secretion of CD11b+ mononuclear cells isolated from bone marrow and of peritoneal macrophages from GPRC6A +/+ (wt) and GPRC6A −/− (ko) mice ( n =5). ( e ) Influence of CaSR and GPRC6A inactivation by transfection with siRNA on IL-1β secretion of THP-1 cells in response to ex[Ca 2+ ]+LPS ( n =3). IBs show inhibition of protein expression of GPRC6A and CaSR in cells transfected with the respective siRNA compared with control siRNA. ( f ) IL-1β secretion of monocytes in response to increasing concentration of Al 3+ with or without LPS ( n =3). ( g ) IL-1β secretion of peritoneal macrophages from GPRC6A +/+ (wt) and GPRC6A −/− (ko) mice in response to 0.9mM Al 3+ plus LPS ( n =3). ( h ) IL-1β secretion of THP-1 cells (control), NLRP3-deficient THP-1 cells (THP1defNLRP3) and ASC-deficient THP-1 cells (THP1defASC) stimulated with 0.9 mM Al 3+ plus LPS, for 16 h ( n =3). ( i ) IL-1β release of monocytes stimulated with different GPCR ligands at the indicated concentration alone (white bars) or with GPCR ligands +LPS (black bars) for 16 h. ( j ) IL-1β release from monocytes stimulated with ex[Ca 2+ ]+LPS in the presence of dimethyl sulfoxide (control) or with the phosphoinositide-specific PLC inhibitor U-73122 (5 μM) in dimethyl sulfoxide ( n =3). ( k ) PLC activity in monocytes stimulated for 16 h with LPS alone or with ex[Ca 2+ ]+LPS ( n =5). ( l ) For [Ca 2+ ] i imaging, monocytes were loaded with the Ca 2+ -sensitive indicator dye Fura-2-AM and subsequently stimulated with ex[Ca 2+ ] (1.7 mM). The increase in [Ca 2+ ] i was inhibited by NPS2143. One representative experiment out of three is shown. ( m ) IL-1β release from monocytes stimulated with ex[Ca 2+ ]+LPS in the presence of increasing concentrations of BAPTA-AM ( n =3). * P <0.05, ** P <0.01 and *** P <0.001, always in comparison with the negative control. Statistical analysis was performed using the two-tailed Student's t -test. All error bars show mean±s.e.m. Full size image To obtain definite proof for the involvement of calcium-sensing GPCRs in mediating ex[Ca 2+ ]-induced inflammasome activation, experiments with GPRC6A −/− mice [15] were performed. IL-1β secretion of monocytic cells from GPRC6A −/− mice in response to ex[Ca 2+ ] ( Fig. 2d ) was significantly reduced compared with those from wt C57BL/6 mice. In vitro differentiated THP-1 cells express both receptors and respond strongly to increased ex[Ca 2+ ] ( Supplementary Fig. S7 ). Transfecting those cells with GPRC6A- or CaSR-specific small interfering RNA (siRNA) resulted in a knockdown of the receptors on the protein level, and reduced significantly the ex[Ca 2+ ]-induced IL-1β production ( Fig. 2e ). Simultaneous knockdown of both receptors inhibited IL-1β secretion by >70% ( Fig. 2e ), indicating that both receptors contribute equally towards ex[Ca 2+ ]-induced IL-1β production. Two alternative agonists of those receptors, Gd 3+ and Al 3+ , also stimulated monocytic IL-1β release in vitro ( Fig. 2f and Supplementary Fig. S8a ). The response to both ligands was reduced in GPRC6A −/− mice ( Fig. 2g and Supplementary Fig. S8b ), and was strictly inflammasome dependent, because IL-1β production was abrogated in both ASC- and NLRP3-deficient THP-1 cells ( Fig. 2h and Supplementary Fig. S8c ). CaSR and GPRC6A are coupled to Gα i and Gα q proteins [12] , [13] , [16] , implicating the cyclic adenosine monophosphate (cAMP) and phosphatidyl–inositol/Ca 2+ signalling pathway in ex[Ca 2+ ]-induced inflammasome activation. The inflammasome-stimulating effect of Gα i /Gα q -coupled GPCR signalling was confirmed with two other ligands binding to Gα i /Gα q -coupled receptors, platelet-activating factor and thrombin, which induced a concentration-dependent increase in IL-1β release in LPS-primed monocytes after 16 h, whereas C5a, Rantes and fMLP (all signalling only via Gα i -protein-coupled receptors) did not ( Fig. 2i ). To test whether Gα q signalling via the phosphatidyl–inositol/Ca 2+ pathway contributes to the inflammasome activation, U-73122, an inhibitor of the phospholipase C (PLC), was added to the cultures and found to effectively abrogate ex[Ca 2+ ]-induced IL-1β release ( Fig. 2j ). Accordingly, PLC activity in monocytes stimulated with ex[Ca 2+ ] was increased, indicating activation of this pathway ( Fig. 2k ). Measurement of cytosolic calcium showed an increase in [Ca 2+ ] i concentration, which occurred immediately after stimulation with ex[Ca 2+ ], and inhibition of calcium-sensing GPCRs by NPS2143 diminished the increase in [Ca 2+ ] i ( Fig. 2l ). Elevating [Ca 2+ ] i using thapsigargin triggered IL-1β release without concomitant increase in IL-1β mRNA expression ( Supplementary Fig. S9 ). Pre-incubation with the cell-permeable Ca 2+ -chelator BAPTA-AM was found to dose-dependently inhibit inflammasome activation by ex[Ca 2+ ] ( Fig. 2m ), thereby corroborating a crucial role of intracellular calcium accumulation, which has also been shown to be required for other inflammasome stimuli [17] , [18] . cAMP induction by direct stimulation of the adenylyl cyclases with forskolin did not induce IL-1β release, the adenylyl cyclase inhibitor SQ22536 had no effect, and no influence of stimulation with increased ex[Ca 2+ ] on intracellular cAMP levels was observed ( Fig. 3a–c ), indicating that Gα i signalling without concomitant Gα q has no role in inflammasome activation. 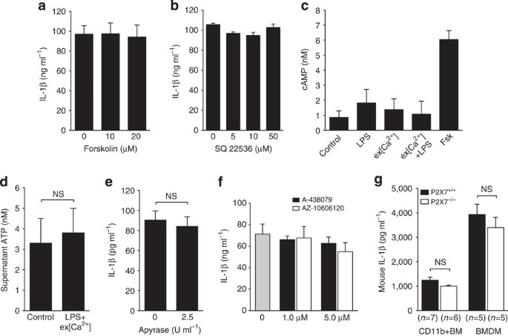Figure 3: The cAMP pathway and extracellular ATP is not involved in ex[Ca2+]-induced inflammasome activation. (a,b) The indicated concentrations of forskolin (a) and of the adenylyl cyclase inhibitor SQ22536 (b) were added to monocyte cultures, and ex[Ca2+] (1.7 mM)-induced IL-1β production was determined (n=3). (c) Intracellular cAMP concentrations in response to ex[Ca2+] (1.7 mM) +LPS (n=3, mean±s.e.m.). Forskolin (Fsk) was used as positive control. All bars show mean±s.e.m. Statistical analysis was performed using a two-tailed Student’st-test, and differences are not statistically significant. (a) ATP concentration in the supernatant of monocytes stimulated with ex[Ca2+] (1.7 mM) +LPS and of unstimulated monocytes (control). (b,c) IL-1β secretion of monocytes stimulated with ex[Ca2+] (1.7 mM) +LPS in the presence of the P2X7 inhibitors A-438079 and AZ-10606120 (b) or apyrase (c) at the indicated concentrations. (d) The ex[Ca2+] +LPS induced IL-1β secretion of CD11b+mononuclear cells isolated from bone marrow and bone marrow-derived macrophages from P2X7+/+and P2X7−/−mice. (a–d) Experiments were performed in triplicates. All bars show mean±s.e.m. Statistical analysis was performed using the two-tailed Student’st-test, and differences are not statistically significant. Figure 3: The cAMP pathway and extracellular ATP is not involved in ex[Ca 2+ ]-induced inflammasome activation. ( a , b ) The indicated concentrations of forskolin ( a ) and of the adenylyl cyclase inhibitor SQ22536 ( b ) were added to monocyte cultures, and ex[Ca 2+ ] (1.7 mM)-induced IL-1β production was determined ( n =3). ( c ) Intracellular cAMP concentrations in response to ex[Ca 2+ ] (1.7 mM) +LPS ( n =3, mean±s.e.m.). Forskolin (Fsk) was used as positive control. All bars show mean±s.e.m. Statistical analysis was performed using a two-tailed Student’s t -test, and differences are not statistically significant. ( a ) ATP concentration in the supernatant of monocytes stimulated with ex[Ca 2+ ] (1.7 mM) +LPS and of unstimulated monocytes (control). ( b , c ) IL-1β secretion of monocytes stimulated with ex[Ca 2+ ] (1.7 mM) +LPS in the presence of the P2X7 inhibitors A-438079 and AZ-10606120 ( b ) or apyrase ( c ) at the indicated concentrations. ( d ) The ex[Ca 2+ ] +LPS induced IL-1β secretion of CD11b+mononuclear cells isolated from bone marrow and bone marrow-derived macrophages from P2X7 +/+ and P2X7 −/− mice. ( a – d ) Experiments were performed in triplicates. All bars show mean±s.e.m. Statistical analysis was performed using the two-tailed Student’s t -test, and differences are not statistically significant. Full size image A known stimulator of the NLRP3 inflammasome is extracellular ATP, which acts as a danger signal when released from dying cells [19] . To exclude autocrine stimulation with ATP via the P2X7 receptor in ex[Ca 2+ ]-induced IL-1β release, we measured ATP levels, added pharmacological P2X7 inhibitors and depleted extracellular ATP using exogenous apyrase. No evidence for autocrine ATP effects was seen ( Fig. 3d–f ). Finally, the ex[Ca 2+ ]-induced IL-1β production of monocytic cells from P2X7 −/− mice did not differ from wt mice ( Fig. 3g ), which all but excludes an influence of endogenously released ATP. Secretory lysosome exocytosis is also not involved in Ca 2+ -induced augmentation of IL-1β release, because no concomitant increase in cathepsin B release was detected ( Supplementary Fig. S10 ). Substantial cell death was also not observed in the monocytes cultures, since the lactate dehydrogenase release was increased only minimally (1.5-fold) in relation to untreated monocytes. ex[Ca 2+ ] induces IL-1α and other proinflammatory cytokines Intracellular calcium accumulation is involved in multiple signalling pathways and can result in diverse cellular outcomes, which prompted us to investigate secretion of other cytokines following stimulation with ex[Ca 2+ ]. Recently, IL-1α has been described to be induced by inflammasome activators [17] . Monocytes stimulated with ex[Ca 2+ ] secreted high concentrations of IL-1α ( Fig. 4a ). Induction of IL-1α was also mediated via CaSR and GPRC6A ( Fig. 4b ), and was absent in THP-1 cells deficient for ASC or NLRP3 ( Fig. 4d ). In addition to IL-1β and IL-1α, monocytes stimulated with ex[Ca 2+ ] were found to secrete IL-6 and TNF ( Supplementary Fig. S11 ). Both cytokines were induced via GPRC6A and CaSR signalling, because secretion was inhibited in GPRC6A −/− mice ( Fig. 4e ) and by Calhex231 and NPS2143 ( Fig. 4f and Supplementary Fig. S11 ), and was dependent on BAPTA-AM-sensitive intracellular calcium accumulation ( Supplementary Fig. S11 ). The lipid mediator prostaglandin E 2 , which has been shown to be induced in macrophages following stimulation with silica crystals [20] , was also detectable in ex[Ca 2+ ]-stimulated monocytes ( Fig. 4g ). 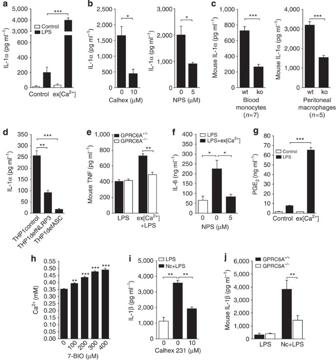Figure 4: Extracellular calcium induces several proinflammatory cytokines and is released from necrotic cells. (a) IL-1α release from unprimed (white bars) and LPS-primed (black bars) monocytes in response to stimulation with ex[Ca2+] (n=3). (b) Influence of the specific inhibitors Calhex231 and NPS2143 on IL-1α secretion of monocytes stimulated with increased ex[Ca2+]+LPS (n=3). (c) ex[Ca2+]-induced IL-1α secretion of CD11b+ mononuclear cells isolated from peripheral blood and of peritoneal macrophages from GPRC6A+/+(wt) and GPRC6A−/−(ko) mice. (d) IL-1α secretion of THP-1 cells (control), NLRP3-deficient THP-1 cells (THP1defNLRP3) and ASC-deficient THP-1 cells (THP1defASC) stimulated with increased ex[Ca2+] concentration and LPS, after 16 h of culture (n=3). (e) Secretion of TNF from LPS-stimulated peritoneal macrophages or from macrophages stimulated with ex[Ca2+]+LPS from GPRC6A+/+(wt) or GPRC6A−/−(ko) mice (n=3). (f) Influence of the specific inhibitor NPS2143 on IL-6 secretion of monocytes stimulated with increased ex[Ca2+]+LPS (n=3). (g) Prostaglandin E2 (PGE2) release from unprimed (white bars) and LPS-primed (black bars) monocytes in response to stimulation with ex[Ca2+] (n=3). (h) Influence of 7-BIO-induced monocyte necrosis on the Ca2+concentration in the supernatant (n=3). (i) IL-1β release from LPS-primed CD14+ monocytes cultured alone (white bars) or co-cultured with necrotic autologous CD4+T cells (black bars) in the absence or presence of the specific inhibitor Calhex231 (n=3). (j) mIL-1β secretion of LPS-primed monocytes from GPRC6A+/+(wt) and GPRC6A−/−(ko) mice cultured alone (LPS) or co-cultured with necrotic autologous CD4+ T cells (Nc+LPS,n=9). All bars show mean±s.e.m. Statistical analysis was performed using the two-tailed Student’st-test. *P<0.05, **P<0.01 and ***P<0.001. Figure 4: Extracellular calcium induces several proinflammatory cytokines and is released from necrotic cells. ( a ) IL-1α release from unprimed (white bars) and LPS-primed (black bars) monocytes in response to stimulation with ex[Ca 2+ ] ( n =3). ( b ) Influence of the specific inhibitors Calhex231 and NPS2143 on IL-1α secretion of monocytes stimulated with increased ex[Ca 2+ ]+LPS ( n =3). ( c ) ex[Ca 2+ ]-induced IL-1α secretion of CD11b+ mononuclear cells isolated from peripheral blood and of peritoneal macrophages from GPRC6A +/+ (wt) and GPRC6A −/− (ko) mice. ( d ) IL-1α secretion of THP-1 cells (control), NLRP3-deficient THP-1 cells (THP1defNLRP3) and ASC-deficient THP-1 cells (THP1defASC) stimulated with increased ex[Ca 2+ ] concentration and LPS, after 16 h of culture ( n =3). ( e ) Secretion of TNF from LPS-stimulated peritoneal macrophages or from macrophages stimulated with ex[Ca 2+ ]+LPS from GPRC6A +/+ (wt) or GPRC6A −/− (ko) mice ( n =3). ( f ) Influence of the specific inhibitor NPS2143 on IL-6 secretion of monocytes stimulated with increased ex[Ca 2+ ]+LPS ( n =3). ( g ) Prostaglandin E2 (PGE 2 ) release from unprimed (white bars) and LPS-primed (black bars) monocytes in response to stimulation with ex[Ca 2+ ] ( n =3). ( h ) Influence of 7-BIO-induced monocyte necrosis on the Ca 2+ concentration in the supernatant ( n =3). ( i ) IL-1β release from LPS-primed CD14+ monocytes cultured alone (white bars) or co-cultured with necrotic autologous CD4+T cells (black bars) in the absence or presence of the specific inhibitor Calhex231 ( n =3). ( j ) mIL-1β secretion of LPS-primed monocytes from GPRC6A +/+ (wt) and GPRC6A −/− (ko) mice cultured alone (LPS) or co-cultured with necrotic autologous CD4+ T cells (Nc+LPS, n =9). All bars show mean±s.e.m. Statistical analysis was performed using the two-tailed Student’s t -test. * P <0.05, ** P <0.01 and *** P <0.001. Full size image Necrotic cells release Ca 2+ and activate the inflammasome Necrotic cells are a potential source of excess extracellular calcium. When necrosis was induced in monocytes with 7-BIO, increased extracellular calcium concentrations were detectable in the supernatant ( Fig. 4h ). Accordingly, co-incubation of monocytes with necrotic cells was found to result in inflammasome activation, which could be inhibited by Calhex231 ( Fig. 4i ). Importantly, inflammasome activation by necrotic cells was significantly inhibited in monocytes from GPRC6A −/− mice ( Fig. 4j ). ex[Ca 2+ ] induces inflammasome activation in vivo To test the in vivo relevance of increased ex[Ca 2+ ], the well-established model of carrageenan-induced footpad swelling was used. In C57BL/6 mice, co-injection of Ca 2+ together with carrageenan resulted in significantly greater footpad swelling compared with carrageenan alone after 1.5 and 4 h ( Fig. 5a ). Similarly, co-injection of Al 3+ or Gd 3+ significantly increased carrageenan-induced footpad swelling ( Fig. 5b–d ). The additional inflammatory effect of co-injected Ca 2+ or Al 3+ was dependent on inflammasome-mediated IL-1β release, because it was reduced both in Caspase-1 −/− and in IL-1R −/− mice ( Fig. 5e–g ). 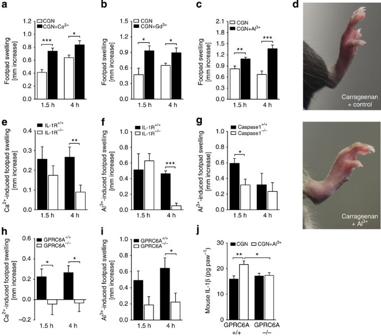Figure 5: CaSR and GPRC6A are involved in inflammatory responsesin vivo. (a–c) Carrageenan (CGN)-induced footpad swelling in C57BL/6 mice with (black bars) or without (white bars) co-injection of Ca2+(n=28) (a), Al3+(n=10) (c,d) or Gd3+(n=6) (b). Bars depict the increase in paw thickness after 1.5 and 4 h compared with baseline. (d) Representative images of CGN-induced footpad swelling after 4 h with (right) or without (left) co-injection of Al3+. (e,f) Ca2+-induced (n=20;e) and Al3+-induced (n=4;f) increase in footpad swelling compared with Carrageenan alone in IL-1R+/+and IL-1R−/−mice after 1.5 and 4 h. (g) Al3+-induced (n=4) increase in footpad swelling compared with Carrageenan alone in Caspase-1+/+and Caspase-1−/−mice after 1.5 and 4 h. (h,i) Ca2+-induced (n=10;h) and Al3+-induced (n=12;i) increase in footpad swelling compared with Carrageenan alone in GPRC6A+/+and GPRC6A−/−mice after 1.5 and 4 h. (j) IL-1β amount in exudats from Carageenan (CGN) or CGN plus Al3+-treated paws from GPRC6A+/+(n=15) and GPRC6A−/−(n=17) mice. All data are expressed as mean±s.e.m. Statistical analysis was performed using a two-tailed Student’st-test,*P<0.05,**P<0.01 and***P<0.001. Figure 5: CaSR and GPRC6A are involved in inflammatory responses in vivo . ( a – c ) Carrageenan (CGN)-induced footpad swelling in C57BL/6 mice with (black bars) or without (white bars) co-injection of Ca 2+ ( n =28) ( a ), Al 3+ ( n =10) ( c , d ) or Gd 3+ ( n =6) ( b ). Bars depict the increase in paw thickness after 1.5 and 4 h compared with baseline. ( d ) Representative images of CGN-induced footpad swelling after 4 h with (right) or without (left) co-injection of Al 3+ . ( e , f ) Ca 2+ -induced ( n =20; e ) and Al 3+ -induced ( n =4; f ) increase in footpad swelling compared with Carrageenan alone in IL-1R +/+ and IL-1R −/− mice after 1.5 and 4 h. ( g ) Al 3+ -induced ( n =4) increase in footpad swelling compared with Carrageenan alone in Caspase-1 +/+ and Caspase-1 −/− mice after 1.5 and 4 h. ( h , i ) Ca 2+ -induced ( n =10; h ) and Al 3+ -induced ( n =12; i ) increase in footpad swelling compared with Carrageenan alone in GPRC6A +/+ and GPRC6A −/− mice after 1.5 and 4 h. ( j ) IL-1β amount in exudats from Carageenan (CGN) or CGN plus Al 3+ -treated paws from GPRC6A +/+ ( n =15) and GPRC6A −/− ( n =17) mice. All data are expressed as mean±s.e.m. Statistical analysis was performed using a two-tailed Student’s t -test, * P <0.05, ** P <0.01 and *** P <0.001. Full size image Final proof for the involvement of GPRC6A in this local inflammatory response was obtained by investigating the model in GPRC6A −/− mice. The results show that both the Ca 2+ - and the Al 3+ -triggered increase in carrageenan-induced footpad swelling was inhibited in the absence of GPRC6A ( Fig. 5h ). Determination of the cytokine content of the injected paws revealed a significant increase in IL-1β in response to Al 3+ , which is absent in paws from GPRC6A −/− mice ( Fig. 5j ). In summary, we provide evidence that increased ex[Ca 2+ ] can activate the NLRP3 inflammasome and Caspase-1, thereby inducing high levels of bioactive IL-1β. Changes in ex[Ca 2+ ] are sensed by monocytes through CaSR signalling [7] , [11] or - as shown here - through GPRC6A signalling, and activate the phosphatidyl–inositol/Ca 2+ pathway, which in turn leads to inflammasome activation. Of note, this is the first report linking GPCR signalling to inflammasome activation. In vivo , ex[Ca 2+ ] has been reported to be increased at sites of infections [5] and ischaemic necrosis [8] , [9] . We propose, therefore, that increased ex[Ca 2+ ] might act as danger-associated molecular pattern (DAMP) by inducing inflammasome activation. In addition, a rise in ex[Ca 2+ ] can result from extrusion to the extracellular fluid during cytosolic calcium signalling [21] , [22] , and the resulting calcium increase in the confined interstitial space can transmit intercellular signalling to neighbouring cells via CaSR [7] or GPRC6A [12] , [13] . Our experiments show that release of Ca 2+ from necrotic cells can also trigger inflammasome activation in neighbouring cells, and that GPRC6A contributes to the transmission of this proinflammatory signal. Consequently, increased ex[Ca 2+ ] could provide a positive feedback loop at sites of inflammation, thereby amplifying secretion of IL-1β and aggravating tissue damage. Consequences of excessive levels of bioactive IL-1β are seen in hereditary and autoimmune diseases, in which IL-1β blockade is clinically effective [23] . We propose that stimulation of monocytes by increased ex[Ca 2+ ] is likely to be of clinical relevance in those and other inflammasome-dependent inflammatory conditions, including atherosclerosis [24] and type 2 diabetes [25] , [26] . While this manuscript was undergoing final review, a related paper was published describing activation of the NLRP3 inflammasome by increased intracellular Ca 2+ via CaSR and decreased cellular cyclic AMP [27] . The study corroborates our finding of an ex[Ca 2+ ]-induced increase in intracellular Ca 2+ , triggering inflammasome activation. In contrast to this study, however, no significant influence of cAMP levels on inflammasone activation was detectable in our system. Most importantly, however, we identified GPRC6A as a second important calcium-sensitive receptor signalling towards inflammasome activation, and also showed the in vivo relevance of this system in an animal model. Antibodies (Abs) and reagents Rabbit-polyclonal anti-Caspase-1 Ab was purchased from Cell Signaling Technology. BAY 61-3606, Calhex231, NPS2143, rabbit-polyclonal anti-IL-1β, rabbit-polyclonal anti-CaSR and anti-GPRC6A Abs and peroxidase-conjugated goat-anti-rabbit secondary Ab were obtained from Santa Cruz Biotechnology. LDH release assay, SQ22536, carrageenan, ATP, thrombin and apyrase were purchased from Sigma-Aldrich. Colchicine, U-73122, fMLP, 4-aminopyridine and forskolin were purchased from Merck. PAF, A-438079 and AZ-10606120 were from Tocris Bioscience. Thapsigargin was from MBL, Tenascin-C from Millipore and Z-WEHD-FMK, C5a and Rantes from R&D Systems. The water-soluble geldanamycin analogue 17-DMAG was purchased from InvivoGen. Human subjects Control subjects were recruited among healthy blood donors. The local ethics committee approved all experiments with human materials, and informed consent was obtained from all subjects. Animal experiments Homozygous genetically deficient B6.129P2-P2rx7tm1Gab/J mice, P2X7 −/− KO mice [28] , B6.129S7-Il1r1tm1Imx/J, NOD.129S2(B6)-Casp1tm1Sesh/LtJ and age-matched wt C57BL/6 and NOD/ShiLtJ controls were purchased from The Jackson Laboratory. GPRC6A −/− mice on a C57BL/6 background were described previously [15] , were used here for in vitro monocyte experiments and in vivo carrageenan-induced footpad swelling and were compared with C57BL/6 wt littermates. Wt or GPRC6A −/− C57BL/6 mice received a subplantar injection of 20 μl of carrageenan (1% w/v) in saline [29] . In some experiments, CaCl 2 (50 mM), Al-lactate (0.3 mg), GdCl 3 (10 mM) or Calhex231 (100 μM) was co-injected. Footpad thickness was assessed by caliper measurement (DigiPlus; Vogel). Measurements were taken immediately before administration of carrageenan and at the indicated time points. The assessment of paw swelling was performed in a double-blind fashion and by the same operator. The increase in paw swelling was calculated by subtracting the initial paw thickness from the paw thickness measured at each time point. For some experiments, mice were euthanized with CO 2 and their hind feet were removed. Paws were put in 250 μl phosphate-buffered saline supplemented with 10% fetal calf serum (FCS) and centrifuged at 1,000 g for 15 min [30] . Mouse IL-1β levels in paw exudates were measured using enzyme-linked immunosorbent assay. Mice were bred and maintained at the animal facilities at the Medizinisch Experimentelles Zentrum, University of Leipzig, Germany. All experiments were approved by and performed according to the institutional guidelines of the animal ethics committee at the University of Leipzig. Cell isolation Human monocytes were isolated as described previously [31] . Bone marrow was obtained by aspirating the femurs of the mice. CD11b+ mononuclear cells were isolated from bone marrow and peripheral blood by positive magnetic separation (Miltenyi Biotech). Peritoneal macrophages were recovered by peritoneal lavage with 5 ml of cold phosphate-buffered saline and used without further separation. Cell culture and calcium titration Monocytes (3 × 10 5 per 200 μl) and THP-1 cells were incubated in RPMI1640 supplemented with 10% heat-inactivated FCS, 2 mM L -glutamine, 100 U ml −1 penicillin and 100 μg ml −1 streptomycin. NLRP3-deficient, ASC-deficient and control THP-1 cells were purchased from InvivoGen. LPS was used at a concentration of 100 ng ml −1 . In the indicated experiments, other TLR ligands (human TLR1-9 Agonist Kit; InvivoGen) were used at following concentrations: Pam3CSK4 (1 μg ml −1 ), heat-killed preparation of Listeria monocytogenes (10 8 cells ml −1 ), Poly(I:C) (10 μg ml −1 ), flagellin (1 μg ml −1 ), FSL1 (1 μg ml −1 ), Imiquimod (1 μg ml −1 ), ssRNA40 (1 μg ml −1 ) and ODN2006 (5 μM). To incubate monocytes in media containing increasing ionized calcium concentration, CaCl 2 was added to the cultures. Final Ca 2+ concentrations in the media were measured after anaerobic sampling (sealed blood gas syringes were completely filled under an CO 2 atmosphere and sealed with caps to avoid loss of CO 2 ) with ABL 730 (Radiometer) by the potentiometric measuring principle, which uses an ion-selective Ca electrode (E733). The amount of CaCl 2 added into the culture medium and the resulting ionized calcium concentration are indicated in Supplementary Table 1 . A final ionized calcium concentration of 1.7 mM was used in the experiments, which was achieved by adding 2.5 mM CaCl 2 to the culture medium. From a concentration of 1.9 mM Ca 2+ in the media, crystals started to precipitate. The IL-1β response using these high Ca 2+ concentrations was not further increased ( Supplementary Fig. S3c ) Undifferentiated THP-1 cells do not express CaSR and GPRC6A on the protein level ( Supplementary Fig. S1 ). To achieve protein expression, THP-1 cells were differentiated for 2 days with phorbol-12-myristate-13-acetate (100 ng ml −1 ). Differentiation with vitamin D3 was not sufficient ( Supplementary Fig. S1 ). Measurement of [Ca 2+ ] i in human monocytes For measurement of [Ca 2+ ] i , human monocytes (1 × 10 6 ) were incubated for 30 min at 37 °C on coverslides with Fura-2/AM (4 μM; Invitrogen) in HBS buffer with 0.2% BSA (Sigma) and 0.6 mM CaCl 2 . In some experiments, 5 μM NPS was added to the cells. Attached cells were rinsed with HBS (0.6 mM or 1.7 mM CaCl 2 ) in a bath chamber and viewed with an inverted epifluorescence microscope (Fluar 10 × /0.5; Axiovert 100 microscope; Carl Zeiss Jena). The fiber-coupled monochromator device (Polychrome V; Till-Photonics) excited fluorescence at alternating wavelength of 340, 358 and 380 nm. Fluorescence emission was imaged with a camera (Sensicam HR; PCO) through a dichroic beam splitter (DCXR-510; Chroma) and a 515-nm long pass filter (OG 515; Schott). Changes of [Ca 2+ ] i were analysed for 200 cells and three different blood donors. Knockdown of CaSR and GPRC6A with siRNA For inactivation of CaSR and GPRC6A, Dharmacon Accell SMARTpool siRNA was applied to THP-1 cells for 4 days before differentiation, as recommended for protein knockdown. For this purpose, THP-1 cells were incubated in RPMI1640 supplemented with 1% heat-inactivated FCS, 2 mM L -glutamine and incubated for 4 days in the presence of 1 μM non-targeting siRNA, CaSR-specific siRNA or GPRC6A-specific siRNA (in each case, a mixture of four different siRNAs). For the final 48 h before detection, THP-1 cells were differentiated with phorbol-12-myristate-13-acetate (100 ng ml −1 ). After 2 days, cells were lysed for western blotting or stimulated with LPS or LPS plus CaCl 2 . Necrotic cells To induce necrosis, cells were exposed to shear stress by aspirating them repeatedly up and down a syringe with a 26-needle gauge. For experiments with human cells, CD4+ T cells from the peripheral blood were used, and for experiment with mouse cells, spleen cells were used. Cell lysis, gel electrophoresis and western blotting Caspase-1 was detected in cell culture supernatants of activated cells, whereas CaSR/GPRC6A was analysed in 3 × 10 6 cells lysed with RIPA buffer. Protein concentrations were determined with a detergent-compatible protein assay (Bio-Rad). Aliquots of the supernatants were incubated in non-reducing Laemmli buffer for 30 min at room temperature (CaSR/GPRC6A) or boiled in reducing Laemmli for 5 min (Caspase-1), and equal amounts of protein were resolved by SDS–PAGE. Gel electrophoresis and western blotting were performed as described previously [30] . Measurement of phosphatidylcholine-specific PLC activity The phosphatidylcholine-specific PLC activity in 1 h-stimulated monocytes was measured using the AmplexRed phosphatidylcholine-specific PLC assay from Invitrogen following the manufacturer’s protocol. Measurement of cytosolic cAMP concentration The cytosolic cAMP concentration in monocytes stimulated for 16 h was determined using the commercially available competition enzyme-linked immunoassay cAMP XP assay (Cell Signaling) following the manufacturer’s protocol. Forskolin was used as a positive control. RNA extraction, cDNA synthesis and quantitive and semi-quantitive PCR Total RNA was prepared using the RNeasy Mini Kit (Qiagen) according to the manufacturer’s protocol. cDNA was transcribed with Multiscribe Reverse Transcriptase (Applied Biosystems) using random hexamers. Quantitative PCR was performed using Taqman Gene Expression Assays for CaSR, GPRC6A and control gene HPRT1 (Applied Biosystems) in the 7500 Real Time PCR System (Applied Biosystems). Results were analysed using 7500 System SDS Software (Applied Biosystems). Semi-quantitative PCR was performed in an Eppendorf Master cycler gradient 5331 using Perkin Elmer PCR reagents. Nlrp3 was amplified using MEP_L_cop32pre-designed primers from Santa Cruz Biotechnology with nested PCR. The first, larger fragment was amplified in 15 cycles and the second, smaller fragment with additional 20 cycles. A 193 bp-fragment of IL-1β was amplified with following primers for 30 cycles (forward 5′-GCATCCAGCTACGAATCTCC-3′, reverse 5′-TCGTTATCCCATGTGTCGAA-3′). PCR fragments were resolved by elecrophoresis on a 2% agarose gel and visualized by ethidium bromide staining. Cytokine measurement Human and mouse IL-1β, TNF and IL-6, mouse IL-1α, (OptEIA; BD Bioscienes), PGE2, human IL-1α (R&D Systems) and human IL-18 (MBL) were measured by commercially available enzyme immunoassay following the manufacturer’s protocol. Statistical analysis For statistical analysis, the software Sigma Stat was used. Before all comparisons, a normality test was performed, which was uniformly passed. Therefore, statistical significance was assessed using the two-tailed Student’s t -test. How to cite this article: Rossol, M. et al . Extracellular Ca 2+ is a danger signal activating the NLRP3 inflammasome through G protein-coupled calcium sensing receptors. Nat. Commun. 3:1329 doi: 10.1038/ncomms2339 (2012).